Serine-7 but not serine-5 phosphorylation primes RNA polymerase II CTD for P-TEFb recognition Phosphorylation of RNA polymerase II carboxy-terminal domain (CTD) in hepta-repeats YSPTSPS regulates eukaryotic transcription. Whereas Ser5 is phosphorylated in the initiation phase, Ser2 phosphorylation marks the elongation state. Here we show that the positive transcription elongation factor P-TEFb is a Ser5 CTD kinase that is unable to create Ser2/Ser5 double phosphorylations, while it exhibits fourfold higher activity on a CTD substrate pre-phosphorylated at Ser7 compared with the consensus hepta-repeat or the YSPTSPK variant. Mass spectrometry reveals an equal number of phosphorylations to the number of hepta-repeats provided, yet the mechanism of phosphorylation is distributive despite the repetitive nature of the substrate. Inhibition of P-TEFb activity is mediated by two regions in Hexim1 that act synergistically on Cdk9 and Cyclin T1. HIV-1 Tat/TAR abrogates Hexim1 inhibition to stimulate transcription of viral genes but does not change the substrate specificity. Together, these results provide insight into the multifaceted pattern of CTD phosphorylation. After transcription initiation, RNA polymerase II (RNAPII) pauses approximately 25–50 nucleotides downstream of the transcription start site because of the action of negative transcription elongation factors [1] . Release from this block requires the positive transcription elongation factor P-TEFb [2] , which is a heterodimer composed of the cyclin-dependent kinase Cdk9 and the regulatory subunit Cyclin T. P-TEFb mediates the transition from transcription initiation to productive elongation of pre-mRNA transcripts by phosphorylation of the carboxy-terminal domain (CTD) of the largest subunit of RNAPII. In humans, the CTD comprises 52 repeats of the consensus sequence Y 1 S 2 P 3 T 4 S 5 P 6 S 7 that exhibits only some variations from the strict consensus towards the C-terminus [3] , [4] , [5] , [6] , [7] . Phosphorylation of Ser5 by Cdk7 and Cdk8 kinases of TFIIH and the mediator complex, respectively, has been described to be concomitant with transcription initiation, whereas Cdk9 of P-TEFb is suggested to phosphorylate Ser2, which marks the elongation phase of transcription [3] , [4] , [5] , [6] , [7] , [8] . In addition, Ser7 of the CTD can also be phosphorylated, which has been linked to small nuclear RNAs (snRNA) transcription and recruitment of the integrator complex [9] , [10] , [11] , [12] , [13] . Whereas some genes, for example, those on CpG islands, can directly proceed to the elongation state by recruiting P-TEFb to RNAPII [14] , genome-wide studies suggest that the majority of genes in higher eukaryotes are under the control of promoter-proximal pausing [15] , [16] , [17] . Studies in budding yeast, whose RNAPII contains 26 hepta-repeats of the consensus CTD sequence, have recently identified gene class-specific CTD phosphorylation patterns and a widespread co-occurrence of such CTD marks at various stages of transcription [18] . Particularly, Ser7 phosphorylation is found early in transcription initiation and retained until transcription termination in all RNAPII-dependent genes. In line with these observations, the dynamics of CTD phosphorylations were found to be not scaled to the gene length but differ among genes with different promoter structures and expression levels [19] . High levels of Ser7 and Ser5 phosphorylations occur at the transcription start site, whereas Ser2 phosphorylation levels increase until they reach their peak about 600–1,000 nucleotides downstream of the start site [20] . These modifications suggest a dual gradient model for increasing Ser2 and decreasing Ser5 phosphorylation across genes that regulate transcription [3] , [4] . In addition to these serine phosphorylations, arginine methylation at one specific residue of the CTD was shown to lead to misregulation of snRNAs as well as small nucleolar RNAs expression [21] . Here we investigated the specificity and activity of P-TEFb for CTD substrates by analytical means as a complementary technique to the use of antibodies raised against designed CTD epitopes. Using various CTD templates we applied mass spectrometry and kinase activity assays for quantification of CTD modifications. Intriguingly, we found that every single hepta-repeat of a CTD substrate can be phosphorylated one time by P-TEFb, though, P-TEFb is unable to phosphorylate a CTD that has been pre-phosphorylated at Ser5 or Ser2 sites. Phosphorylation of Ser7 instead results in a fourfold higher catalytic activity for such modified templates. Inhibition of P-TEFb activity by its cellular regulation factor Hexim1 requires two distinct regions, a central PYNT motif and a C-terminal cyclin T-binding domain (TBD). Both regions act synergistically on the P-TEFb subunits Cdk9 and Cyclin T1, but are ineffective independently. Addition of 7SK snRNA to Hexim1 significantly increases this inhibitory effect. The HIV-1 Tat–TAR complex abrogates Hexim1 inhibition on P-TEFb to stimulate transcription of viral genes but does not change the substrate specificity. These observations provide insights into the kinetics and substrate specificity of the transcription elongation factor P-TEFb, its phosphorylation signature on the RNAPII CTD and regulation by cellular factors. The number of CTD phosphorylations equals the hepta-repeats We set up an in vitro phosphorylation assay using recombinant P-TEFb and CTD substrates containing 5 to 13 consensus hepta-repeats or all 52 hepta-repeats of human wild-type CTD (Methods). The homogeneity and functional integrity of the P-TEFb complex was assayed by mass spectrometry, size exclusion chromatography and radioactive filter-binding experiments to confirm its catalytic activity ( Supplementary Fig. S1 ). At a temperature of 30 °C, saturation of the CTD phosphorylation reaction was achieved within several hours of incubation, using twofold molar excess of the co-substrate ATP over the concentration of CTD substrate multiplied by the number of hepta-repeats contained in the substrate ( Fig. 1a ). The increasing phosphorylation status of a glutathione S -transferase (GST)–CTD fusion protein and the gain in mass upon each phosphorylation is also visible as retained migration behaviour in SDS-polyacrylamide gel electrophoresis (PAGE) analysis ( Fig. 1b ). 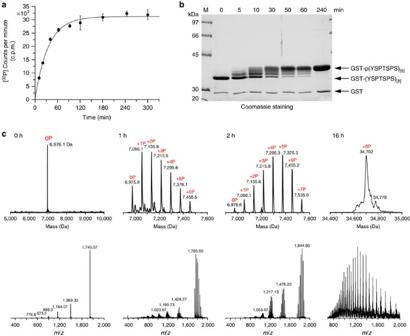Figure 1: P-TEFb phosphorylates the CTD in a distributive mechanism equally to the number of hepta-repeats. (a) Time course of CTD phosphorylation in a P-TEFb kinase assay. A GST–CTD[13]fusion protein containing 13 hepta-repeats (10 μM) was incubated with 0.1 μM P-TEFb and 300 μM [32P]-γ-labelled ATP. Saturation of the phosphorylation reaction was achieved within 3 h. Data represent the mean±range from two independent experiments. (b) SDS–PAGE analysis of CTD phosphorylation by P-TEFb. At concentrations of 0.1 μM P-TEFb, 100 μM GST–CTD[8]and 3 mM ATP the substrate was fully phosphorylated after 4 h at 30 °C. (c) ESI-MS analysis of CTD phosphorylation in a time course experiment. A CTD peptide containing eight hepta-repeats was used as P-TEFb substrate. Shown are time points at the beginning and after 1, 2 and 16 h of the reaction. For the last time point, a GST–CTD[8]substrate was used for better ionization properties in the ESI-MS analysis. Figure 1: P-TEFb phosphorylates the CTD in a distributive mechanism equally to the number of hepta-repeats. ( a ) Time course of CTD phosphorylation in a P-TEFb kinase assay. A GST–CTD [13] fusion protein containing 13 hepta-repeats (10 μM) was incubated with 0.1 μM P-TEFb and 300 μM [ 32 P]-γ-labelled ATP. Saturation of the phosphorylation reaction was achieved within 3 h. Data represent the mean±range from two independent experiments. ( b ) SDS–PAGE analysis of CTD phosphorylation by P-TEFb. At concentrations of 0.1 μM P-TEFb, 100 μM GST–CTD [8] and 3 mM ATP the substrate was fully phosphorylated after 4 h at 30 °C. ( c ) ESI-MS analysis of CTD phosphorylation in a time course experiment. A CTD peptide containing eight hepta-repeats was used as P-TEFb substrate. Shown are time points at the beginning and after 1, 2 and 16 h of the reaction. For the last time point, a GST–CTD [8] substrate was used for better ionization properties in the ESI-MS analysis. Full size image For a quantitative analysis, we used electrospray ionization mass spectrometry (ESI-MS) to determine the number of phosphorylation events at various time points. Towards the endpoint of the reaction under saturating conditions, the number of phosphorylations as determined by mass spectrometry equals the number of hepta-repeats provided in the CTD substrate ( Fig. 1c ). Although this result may seem trivial, it confirms a high specificity of P-TEFb for the CTD substrate given that three canonical serines are present in each hepta-repeat, two of them as the preferred Ser-Pro recognition motif for Cdk family kinase phosphorylation [22] , [23] . It also indicates that a continuous phosphorylation signature can be achieved by P-TEFb, leaving no gaps in the modification pattern of the CTD hepta-repeat structure. These results were confirmed by the potent phosphorylation of a full-length CTD containing all 52 hepta-repeats including the acidic C-terminus ( Supplementary Fig. S2 ). Although the highly negatively charged CTD was not accessible to mass spectrometry analysis, the large band shift upon phosphorylation and the passage into saturation suggest full phosphorylation of the substrate. A distributive CTD phosphorylation mechanism by PTefb Mass spectra recorded in the course of the reaction provided additional insights into the phosphorylation mechanism ( Fig. 1c ). Assuming that all phosphorylated CTD substrates are similarly susceptible to ionization, the phosphorylation spectra recorded represent a histogram of the number of molecules containing no, one, two etc., phosphorylations, albeit without any information about the spatial arrangement of these modifications on the periodic template. The asymmetric distribution of the mass spectra recorded at 1 and 2 h after reaction start indicate a binominal distribution function with two boundaries, '0' and '8' in this experiment. From the statistics of mass increase it can be concluded that the mechanism of CTD phosphorylation by P-TEFb is distributive, rather than processive, as might be suspected from the repetitive nature of the substrate. An illustration of a distributive versus a processive reaction mechanism on a periodic matrix as the CTD and the corresponding histograms of mass distributions are shown in Supplementary Fig. S3 . However, it cannot be excluded that a consecutive phosphorylation mechanism applies to the mode of P-TEFb action, meaning that once a first phosphorylation mark has been set on a substrate template, the following (upstream or downstream) hepta-repeat will be phosphorylated preferentially due to an increased recognition affinity. CTD-pSer7 is the preferred P-TEFb substrate To analyse the preference of P-TEFb for particular sequence compositions and phosphorylation signatures, we designed a series of CTD peptides, each containing three hepta-repeats ( Fig. 2a ). The peptides contained the unmodified consensus CTD sequence (cons. CTD [3] ), phosphoryl groups at Ser2, Ser5 or Ser7 throughout (pS2-CTD [3] , pS5-CTD [3] and pS7-CTD [3] , respectively) or lysines at position 7 (K7-CTD [3] ). The hepta-repeat sequence YSPTSPK is indeed the prevailing alteration from the consensus CTD in higher eukaryotes, occurring eight times in human RNAPII. The peptides were marked at the C-terminus with a double arginine motif separated by a polyethylene glycol spacer for better ionization properties in the ESI-MS analysis. 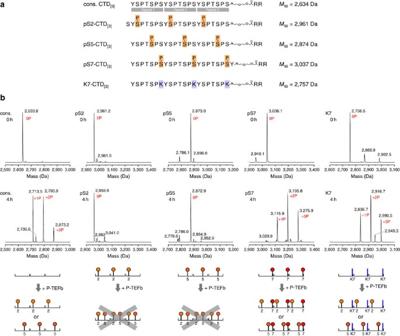Figure 2: P-TEFb is unable to phosphorylate a CTD pre-phosphorylated at Ser5 or Ser2. (a) Design of CTD substrate peptides used for kinetic and ESI-MS analyses. Peptides contained three consensus hepta-repeats with either no modification (cons. CTD[3]), a phosphorylation mark continuously set at Ser2 (pS2-CTD[3]), at Ser5 (pS5-CTD[3]), at Ser7 (pS7-CTD[3]) or a lysine residue at position 7 (K7-CTD[3]). (b) ESI-MS analyses of CTD peptides before and after 4 h of incubation with P-TEFb. For the pS2-CTD[3]and pS5-CTD[3]templates no phosphorylation by P-TEFb occurred, while pS7-CTD[3]got readily phosphorylated. Cartoons displaying the possible phosphorylation patterns are shown at the bottom. Figure 2: P-TEFb is unable to phosphorylate a CTD pre-phosphorylated at Ser5 or Ser2. ( a ) Design of CTD substrate peptides used for kinetic and ESI-MS analyses. Peptides contained three consensus hepta-repeats with either no modification (cons. CTD [3] ), a phosphorylation mark continuously set at Ser2 (pS2-CTD [3] ), at Ser5 (pS5-CTD [3] ), at Ser7 (pS7-CTD [3] ) or a lysine residue at position 7 (K7-CTD [3] ). ( b ) ESI-MS analyses of CTD peptides before and after 4 h of incubation with P-TEFb. For the pS2-CTD [3] and pS5-CTD [3] templates no phosphorylation by P-TEFb occurred, while pS7-CTD [3] got readily phosphorylated. Cartoons displaying the possible phosphorylation patterns are shown at the bottom. Full size image After 4 h incubation with P-TEFb, the consensus CTD substrate showed up to three phosphorylations corresponding to the three hepta-repeats provided as indicated by mass increases ( Fig. 2b ). Intriguingly, we found that P-TEFb is unable to phosphorylate a CTD substrate that contained complete phosphorylation at Ser5. Likewise, a peptide-containing phosphoryl group at Ser2 was not phosphorylated after 4 h incubation. In sharp contrast, P-TEFb readily phosphorylated a CTD template pre-phosphorylated at position Ser7. The alternate K7 hepta-repeats again were phosphorylated, while phosphorylation of either Tyr1 or the recently identified Thr4 residues [24] , [25] abrogated P-TEFb activity for these pre-modified substrates ( Supplementary Fig. S4 ). Notably, a similar recognition preference for the phosphorylation of cons. CTD, pS7-CTD and K7-CTD but not pS2- and pS5-CTD was seen for native P-TEFb that contained besides full-length Cdk9 also full-length CycT1 ( Supplementary Fig. S5 ). Kinetics of P-TEFb-mediated CTD phosphorylations From a time course of the reaction, a K cat / K M value of 2.15×10 4 M −1 s −1 was determined for the pS7-CTD [3] substrate, whereas P-TEFb showed a K cat / K M value of 5.5×10 3 M −1 s −1 for the consensus CTD using an enzyme concentration of 0.1 μM ( Fig. 3 ). Surprisingly, the CTD sequence modified with a lysine residue at position 7 exhibited with a K cat / K M value of 5.2×10 3 M −1 s −1 similar substrate susceptibility for P-TEFb as the consensus sequence. Using longer CTD templates of 9 or 13 repeats uniformly modified with lysines at position 7, as found, for example, in Plasmodium falciparum [5] , we noticed, however, a retarded phosphorylation activity of P-TEFb. Such effect could result from a changed accessibility of the serines, possibly caused by ionic interactions between lysines and phosphate groups. 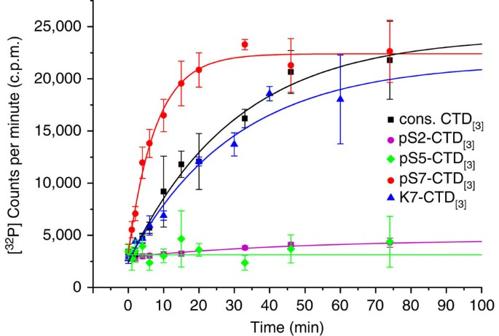Figure 3: Kinetics of P-TEFb-mediated phosphorylation of different CTD substrates. P-TEFb exhibits a fourfold higher enzymatic activity for a CTD substrate phosphorylated at Ser7 (pS7-CTD[3]) compared with the unmodified consensus sequence (cons. CTD[3]). A CTD-containing lysine at position 7 (K7-CTD[3]) showed a similar susceptibility for P-TEFb as the consensus sequence, whereas Ser2 and Ser5 pre-phosphorylated substrates (pS2-CTD[3]and pS5-CTD[3]) were abrogated for additional phosphorylation modifications by P-TEFb. All data were reported as the mean±s.d. from three independent experiments. Figure 3: Kinetics of P-TEFb-mediated phosphorylation of different CTD substrates. P-TEFb exhibits a fourfold higher enzymatic activity for a CTD substrate phosphorylated at Ser7 (pS7-CTD [3] ) compared with the unmodified consensus sequence (cons. CTD [3] ). A CTD-containing lysine at position 7 (K7-CTD [3] ) showed a similar susceptibility for P-TEFb as the consensus sequence, whereas Ser2 and Ser5 pre-phosphorylated substrates (pS2-CTD [3] and pS5-CTD [3] ) were abrogated for additional phosphorylation modifications by P-TEFb. All data were reported as the mean±s.d. from three independent experiments. Full size image Reverse kinase order does not induce double phosphorylations As an alternative progression of P-TEFb function, we thought to test Cdk kinase activities in reverse order such that after incubation with P-TEFb the CTD substrate was subjected to Cdk7 to test for higher phosphorylation modes. Whereas the Cdk7/CycH/MAT1 subunits of the TFIIH complex efficiently phosphorylated the unmodified CTD in control experiments, no indication for additional phosphorylations on a template that was first incubated with P-TEFb was observed ( Supplementary Fig. S6 ). Similarly, no additional phosphorylation marks were seen with Cdk7 for a P-TEFb pre-phosphorylated CTD-containing lysines at position 7 throughout. As before, the maximum number of phosphorylations equals the number of hepta-repeats presented. These results can be seen as indirect evidence that neither Cdk7 nor Cdk9 phosphorylates Ser7 to a significant extent as otherwise the number of phosphorylations should be higher than the number of hepta-repeats provided. P-TEFb is a Ser5 CTD kinase Following the observation that P-TEFb neither phosphorylated a CTD template that contained continuous Ser5 nor Ser2 phosphorylations, we thought to re-analyse its substrate specificity by analytical means. Four different approaches were used to challenge the dogma of Ser2 phosphorylation by P-TEFb: alanine mutagenesis, western blot analyses, size constraints with either one or two alternating phosphorylation sites and peptide modifications by serine acetylation. Using a similar design as described above, two CTD peptides were generated that contained alanine at either position 2 or 5 throughout ( Fig. 4a ). Yet, although the Ala2 peptide was phosphorylated by P-TEFb up to three times, no significant phosphorylation was seen for the Ala5 peptide ( Fig. 4b ). Western blot analysis using anti-phospho-CTD-specific antibodies raised against either pSer2, pSer5 or pSer7 phosphorylations showed a prevalence of Ser5 phosphorylation by P-TEFb on the GST full-length CTD substrate ( Fig. 4c ). Some Ser7 phosphorylations were also detected, whereas virtually no Ser2 phosphorylation marks were seen on the native substrate. Next, a 13-mer CTD peptide containing Ser2 at its centre was synthesized, harbouring thus only one bona fide Ser2 site but two Ser5 positions. After 4 h incubation with P-TEFb, up to two additional phosphorylations on the substrate template were detected by quantitative high-performance liquid chromatography (HPLC) analysis ( Fig. 4d ). In contrast, only one additional phosphorylation was achieved for a peptide containing Ser5 at its centre ( Fig. 4e ). To assign the site of phosphorylation in more detail, again a 13-mer peptide was generated but with the central Ser2 residue acetylated in order to prevent its phosphorylation. Again up to two phosphorylations were seen by analytical HPLC upon incubation with P-TEFb ( Fig. 4f ). The same peptide stretch containing Ser5 acetylation but not Ser2 showed instead a majority of remaining unphosphorylated peptide, whereas only a minor fraction with one additional phosphorylation was detected ( Fig. 4g ). These data suggest that P-TEFb preferentially phosphorylates Ser5 on a RNAPII CTD substrate, whereas a small ambiguity for Ser2 phosphorylation may remain. 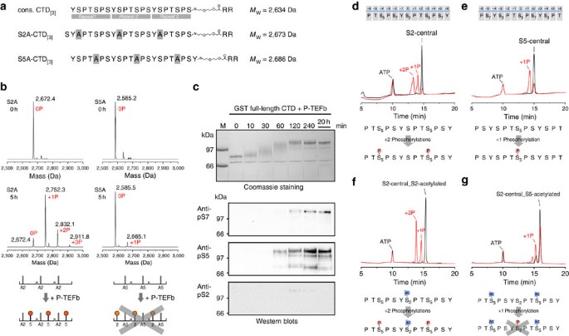Figure 4: P-TEFb is a Ser5 CTD kinase. (a) Design of CTD substrate peptides containing alanine mutations at either position 2 or 5 in each repeat. (b) ESI-MS analyses after 5 h incubation with P-TEFb showed that the S2A CTD mutant is still susceptible as P-TEFb substrate while no phosphorylation occurred for the S5A mutant. (c) Coomassie staining and western blot analysis of P-TEFb-mediated CTD phosphorylation. Full-length human CTD containing all 52 hepta-repeats was applied in time course experiments. Phospho-serine-directed antibodies reveal a preference of P-TEFb for Ser5 phosphorylation. (d) HPLC analysis on a 13-mer CTD peptide with Ser2 at its centre showed up to two phosphorylations by P-TEFb. (e) The same peptide length with Ser5 at its centre showed only one phosphorylation. (f) As control, the same peptide sequence as indwas synthesized with the central Ser2 residue being acetylated to prevent its phosphorylation. Again, two additional phosphorylations were achieved after P-TEFb incubation. (g) The same peptide sequence as indwas synthesized with the two distant Ser5 residues being acetylated. Only a minor fraction was detected that contained one additional phosphorylation. Figure 4: P-TEFb is a Ser5 CTD kinase. ( a ) Design of CTD substrate peptides containing alanine mutations at either position 2 or 5 in each repeat. ( b ) ESI-MS analyses after 5 h incubation with P-TEFb showed that the S2A CTD mutant is still susceptible as P-TEFb substrate while no phosphorylation occurred for the S5A mutant. ( c ) Coomassie staining and western blot analysis of P-TEFb-mediated CTD phosphorylation. Full-length human CTD containing all 52 hepta-repeats was applied in time course experiments. Phospho-serine-directed antibodies reveal a preference of P-TEFb for Ser5 phosphorylation. ( d ) HPLC analysis on a 13-mer CTD peptide with Ser2 at its centre showed up to two phosphorylations by P-TEFb. ( e ) The same peptide length with Ser5 at its centre showed only one phosphorylation. ( f ) As control, the same peptide sequence as in d was synthesized with the central Ser2 residue being acetylated to prevent its phosphorylation. Again, two additional phosphorylations were achieved after P-TEFb incubation. ( g ) The same peptide sequence as in d was synthesized with the two distant Ser5 residues being acetylated. Only a minor fraction was detected that contained one additional phosphorylation. Full size image In a second set of experiments, the directionality of CTD phosphorylation by P-TEFb was addressed. Using CTD substrate peptides of three hepta-repeats that contained only one Ser5 phosphorylation at either end of the template ( Fig. 5a ), we found that P-TEFb exhibited an almost fourfold higher catalytic activity for the substrate when the phosphorylation mark was placed at the C-terminus ( Fig. 5b,c ). Such differences in the amino- or carboxy-terminal extension kinetics to pre-existing phosphorylation sites could indicate a preferred directionality of the enzyme during the phosphorylation reaction. 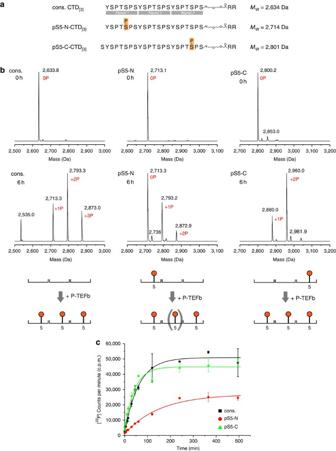Figure 5: Kinetics of P-TEFb activity on partially pre-phosphorylated CTD substrates. (a) Design of CTD substrate peptides containing a Ser5 phosphorylation mark in either the N- or C-terminal hepta-repeat. The peptides were used for mass spectrometry and kinetic analyses. (b) ESI-MS analyses after 6 h incubation time with P-TEFb revealed a majority of two additional phosphorylations for the CTD substrate when the pSer5 mark was set in the C-terminal repeat (pS5-C-CTD[3]), whereas only one additional phosphorylation prevailed after the same incubation time when the Ser5 phosphorylation mark was set in the N-terminal repeat (pS5-N-CTD[3]). (c) Kinetic analysis showed a fourfold higher catalytic activity of P-TEFb for a substrate containing a C-terminal Ser5 phosphorylation mark compared with the reversed order. At a concentration of 0.2 μM P-TEFb, aKcat/KMvalue of 4.1×103M−1s−1was determined for pS5-C-CTD[3]compared with 1.1×103M−1s−1for pS5-C-CTD[3]and 2.8×103M−1s−1for the consensus CTD substrate. Data are the mean of two independent experiments; bars indicate the range. Figure 5: Kinetics of P-TEFb activity on partially pre-phosphorylated CTD substrates. ( a ) Design of CTD substrate peptides containing a Ser5 phosphorylation mark in either the N- or C-terminal hepta-repeat. The peptides were used for mass spectrometry and kinetic analyses. ( b ) ESI-MS analyses after 6 h incubation time with P-TEFb revealed a majority of two additional phosphorylations for the CTD substrate when the pSer5 mark was set in the C-terminal repeat (pS5-C-CTD [3] ), whereas only one additional phosphorylation prevailed after the same incubation time when the Ser5 phosphorylation mark was set in the N-terminal repeat (pS5-N-CTD [3] ). ( c ) Kinetic analysis showed a fourfold higher catalytic activity of P-TEFb for a substrate containing a C-terminal Ser5 phosphorylation mark compared with the reversed order. At a concentration of 0.2 μM P-TEFb, a K cat / K M value of 4.1×10 3 M −1 s −1 was determined for pS5-C-CTD [3] compared with 1.1×10 3 M −1 s −1 for pS5-C-CTD [3] and 2.8×10 3 M −1 s −1 for the consensus CTD substrate. Data are the mean of two independent experiments; bars indicate the range. Full size image Two regions in Hexim1 are required for P-TEFb inhibition The cellular protein Hexim1 is an inhibitor of P-TEFb activity by an as yet unknown mechanism [2] . Using the in vitro kinase assay, we set out to determine the molecular requirements of P-TEFb inhibition quantitatively. Under standard conditions, 0.1 μM P-TEFb was mixed with 100 μM GST–CTD [8] and 100 μM ATP and incubated for 10 min before the solution was spotted onto filter paper and the reaction stopped by immersing the filter paper in phosphoric acid. Under these conditions full-length Hexim1 at a concentration of 2.5 μM inhibited P-TEFb activity to 28% without addition of 7SK snRNA. In contrast, 2.5 μM of the 332 nucleotides encompassing 7SK showed no effect on P-TEFb, a result also obtained with the 66-mer 5′-hairpin finger that was previously identified to interact with Hexim1 (ref. 26 ; Fig. 6a ). The addition of a Hexim1/7SK snRNA complex instead inhibited P-TEFb activity almost completely (3%), as did flavopiridol (2%). These results confirm a role of 7SK snRNA as a scaffold for Hexim1-mediated P-TEFb inhibition. 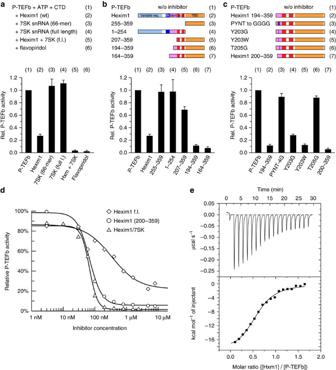Figure 6: Inhibition of P-TEFb requires two distinct motifs in different domains of Hexim1. (a) Effect of Hexim1 and 7SK snRNA on the kinase activity of P-TEFb. The inhibitory effect of full-length Hexim1 was significantly increased by 7SK, although 7SK showed no influence on its own. (b) Mapping of the functional relevant sites in Hexim1 for P-TEFb inhibition. Although the Cyclin T-binding domain (TBD) is required for P-TEFb recognition, residues between 194 and 206 are required for Cdk9 inhibition. (c) Mutation of T205G within a highly conserved PYNT motif in Hexim1 194–359 abrogated its inhibitory effect on P-TEFb activity. Mutation of Y203G or Y203W instead potently retained the inhibitory function of Hexim1. Data ina–care the mean±s.d. from three independent experiments. (d) A concentration series of Hexim1 inhibitor constructs at 100 nM P-TEFb concentration revealed IC50values of 339 nM for full-length Hexim1, 67 nM for the complex of full-length Hexim1 and 7SK snRNA, and 67 nM for N-terminally truncated Hexim1 variant 200–359. (e) Isothermal titration calorimetry measurement of P-TEFb with Hexim1 194–359 indicated a dissociation constant of 0.3 μM. Figure 6: Inhibition of P-TEFb requires two distinct motifs in different domains of Hexim1. ( a ) Effect of Hexim1 and 7SK snRNA on the kinase activity of P-TEFb. The inhibitory effect of full-length Hexim1 was significantly increased by 7SK, although 7SK showed no influence on its own. ( b ) Mapping of the functional relevant sites in Hexim1 for P-TEFb inhibition. Although the Cyclin T-binding domain (TBD) is required for P-TEFb recognition, residues between 194 and 206 are required for Cdk9 inhibition. ( c ) Mutation of T205G within a highly conserved PYNT motif in Hexim1 194–359 abrogated its inhibitory effect on P-TEFb activity. Mutation of Y203G or Y203W instead potently retained the inhibitory function of Hexim1. Data in a – c are the mean±s.d. from three independent experiments. ( d ) A concentration series of Hexim1 inhibitor constructs at 100 nM P-TEFb concentration revealed IC 50 values of 339 nM for full-length Hexim1, 67 nM for the complex of full-length Hexim1 and 7SK snRNA, and 67 nM for N-terminally truncated Hexim1 variant 200–359. ( e ) Isothermal titration calorimetry measurement of P-TEFb with Hexim1 194–359 indicated a dissociation constant of 0.3 μM. Full size image We next fragmented Hexim1 in the C-terminal Cyclin TBD (residues 255–359) and the remaining regulatory segment 1–254. Interestingly, neither fragment inhibited P-TEFb activity ( Fig. 6b ), although the TBD was shown before to interact with CycT1 at a site required in the Cdk2–CycA complex for substrate recognition [27] . Further N-terminal elongations of the TBD revealed a marked increase in the inhibitory potential of a construct starting at position 194 compared with position 207, suggesting that residues 194–206 are necessary for the inhibitory function of Hexim1 ( Fig. 6b ). Point mutations identified a PYNT motif at position 202 as the inhibitory region of Hexim1, in accordance with previous studies in vivo [28] . The largest effect, however, was not contributed by Y203, as suggested in analogy to Cdk2-CycA inhibition by p27 Kip , but by T205, whose mutation to glycine almost fully abrogated the inhibitory potential of Hexim1 (88% relative activity, Fig. 6c ). The homogeneity of the various Hexim1 mutant proteins tested is shown in Supplementary Fig. S7 . The inhibitory effect of N-terminally truncated Hexim1 200–359 was indeed as potent as full-length Hexim1 bound to 7SK snRNA, supporting previous observations that the N-terminal part of Hexim1 could be self-inhibitory [29] . At concentrations of 100 nM P-TEFb, half-maximal inhibitory concentration (IC 50 ) values of 67 nM for Hexim1 200–359 and 67 nM for Hexim1/7SK, respectively, were determined compared with an IC 50 of 339 nM for full-length Hexim1 ( Fig. 6d ). In binding experiments using isothermal titration calorimetry (ITC), the T205G mutation reduced the affinity of Hexim1 for P-TEFb about sevenfold to the portion of the Hexim1 TBD–CycT1 interaction ( Table 1 ). These results support the synergistic contribution of the central PYNT motif in Hexim1 to the C-terminal TBD, which are required for Cdk9 kinase inhibition and CycT1 binding ( Fig. 6e and Table 1 ). Table 1 Thermodynamic analysis of Hexim1 binding to P-TEFb (Cdk9/CycT1) or CycT1 alone determined by isothermal titration calorimetry. Full size table HIV-1 Tat/TAR does not change P-TEFb phosphorylations Addition of either HIV-1 Tat or the HIV-1 Tat/TAR ribonucleoprotein complex in increasing amounts to P-TEFb/Hexim1 led to recovery of the kinase activity in the substrate activity assay ( Fig. 7a ). This effect is supposed to occur by displacement of Hexim1 from its binding site on CycT1, as no ternary complex between these two P-TEFb regulating proteins with CycT1 is formed [30] , [31] . An indication for a change or weakening of the P-TEFb substrate specificity towards both Ser2 and Ser5 phosphorylation [32] , [33] , for example, by means of increasing numbers of phosphorylation, was not observed. Addition of Tat or Tat/TAR led to an approximately twofold higher activity of P-TEFb to a consensus CTD substrate, though the number of phosphorylations remained unchanged ( Fig. 7b and Supplementary Figs S5 and S8 ). This result was confirmed on the full-length CTD where the viral protein–RNA complex did not induce a super-shift in the migration pattern of the phosphorylated substrate ( Fig. 7c ). 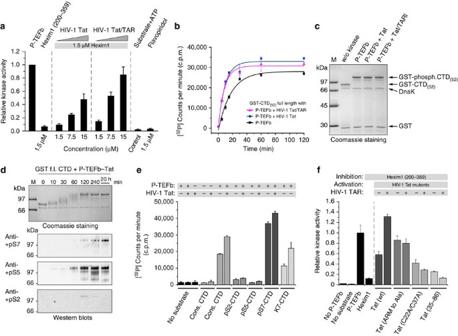Figure 7: HIV-1 Tat/TAR overcomes P-TEFb inhibition of Hexim1 but does not change its substrate specificity. (a) The kinase activity of 0.1 μM P-TEFb using GST–CTD[8]substrate and radioactive-labelled ATP co-substrate was measured after 10 min incubation (left column). Inhibition of P-TEFb activity by Hexim1 200–359 led to a reduction of kinase activity to 6% (second column). Addition of either HIV-1 Tat or the preformed HIV-1 Tat/TAR complex in increasing concentrations recovered P-TEFb activity (central columns). As controls, substrate plus ATP without P-TEFb or with P-TEFb with flavopiridol were measured (right columns). (b) Kinetics of Tat/TAR-stimulated P-TEFb activity in the absence of Hexim1. Full-length GST–CTD[52]at 2.5 μM concentration was incubated with 2 mM ATP and 0.2 μM P-TEFb. HIV-1 Tat 1–86 or Tat/TAR was added before the reaction at concentrations of 2 μM. The specific activitiesKcat/KMwere determined to 4.7×103M−1s−1for P-TEFb, 8.8×103M−1s−1for P-TEFb–Tat, and 9.6×103M−1s−1for P-TEFb with Tat/TAR. (c) SDS–PAGE analysis of P-TEFb phosphorylated full-length CTD in the presence or absence of Tat or Tat/TAR showed no increase in the migration pattern. (d) Western blot analysis of P-TEFb–Tat-mediated CTD phosphorylation revealed prevalence for Ser5 phosphorylation. (e) The substrate specificity of P-TEFb on synthesized CTD peptides remained unchanged in the presence of HIV-1 Tat. The phosphorylation efficacy was monitored after 15 min. (f) Effects of Tat mutations on the recovery of P-TEFb activity in the presence of Hexim1. To a concentration of 0.1 μM P-TEFb, 100 μM GST–CTD and 1 mM ATP, a concentration of 1.5 μM Hexim1 was added for inhibition and 15 μM Tat or Tat/TAR for activation. Disruption of the intermolecular zinc-finger formation by mutation C22A/C37A or N-terminal truncation 35–86 significantly reduced the ability of Tat to activate P-TEFb. Data shown ina,b,eandfare the mean±s.d. from three independent experiments. Figure 7: HIV-1 Tat/TAR overcomes P-TEFb inhibition of Hexim1 but does not change its substrate specificity. ( a ) The kinase activity of 0.1 μM P-TEFb using GST–CTD [8] substrate and radioactive-labelled ATP co-substrate was measured after 10 min incubation (left column). Inhibition of P-TEFb activity by Hexim1 200–359 led to a reduction of kinase activity to 6% (second column). Addition of either HIV-1 Tat or the preformed HIV-1 Tat/TAR complex in increasing concentrations recovered P-TEFb activity (central columns). As controls, substrate plus ATP without P-TEFb or with P-TEFb with flavopiridol were measured (right columns). ( b ) Kinetics of Tat/TAR-stimulated P-TEFb activity in the absence of Hexim1. Full-length GST–CTD [52] at 2.5 μM concentration was incubated with 2 mM ATP and 0.2 μM P-TEFb. HIV-1 Tat 1–86 or Tat/TAR was added before the reaction at concentrations of 2 μM. The specific activities K cat / K M were determined to 4.7×10 3 M −1 s −1 for P-TEFb, 8.8×10 3 M −1 s −1 for P-TEFb–Tat, and 9.6×10 3 M −1 s −1 for P-TEFb with Tat/TAR. ( c ) SDS–PAGE analysis of P-TEFb phosphorylated full-length CTD in the presence or absence of Tat or Tat/TAR showed no increase in the migration pattern. ( d ) Western blot analysis of P-TEFb–Tat-mediated CTD phosphorylation revealed prevalence for Ser5 phosphorylation. ( e ) The substrate specificity of P-TEFb on synthesized CTD peptides remained unchanged in the presence of HIV-1 Tat. The phosphorylation efficacy was monitored after 15 min. ( f ) Effects of Tat mutations on the recovery of P-TEFb activity in the presence of Hexim1. To a concentration of 0.1 μM P-TEFb, 100 μM GST–CTD and 1 mM ATP, a concentration of 1.5 μM Hexim1 was added for inhibition and 15 μM Tat or Tat/TAR for activation. Disruption of the intermolecular zinc-finger formation by mutation C22A/C37A or N-terminal truncation 35–86 significantly reduced the ability of Tat to activate P-TEFb. Data shown in a , b , e and f are the mean±s.d. from three independent experiments. Full size image The substrate specificity of P-TEFb when bound to Tat remained unaltered compared with P-TEFb alone. First, western blot analysis revealed the same prevalence of P-TEFb–Tat for Ser5 phosphorylation as seen with P-TEFb alone ( Fig. 7d and Supplementary Fig. S9 ). Likewise, using the synthesized CTD peptide library in a radioactive kinase assay, we found that the P-TEFb–Tat complex showed again a higher activity for a CTD substrate pre-phosphorylated at Ser7 compared with the consensus CTD sequence, whereas Ser2 or Ser5 pre-phosphorylations abrogated their recognition as potential substrate ( Fig. 7e ). After 15 min incubation, phosphorylation numbers were always increased in the presence of Tat, whereas control measurements confirmed that Tat did not act itself as a substrate. The moderate increase in P-TEFb activity could result, for example, from advanced ionic interactions of basic residues in Tat with the negatively charged substrate. In addition, the effect of Tat mutants that were described to specifically influence Tat functions [34] were analysed for their ability to recover P-TEFb activity from inhibition by Hexim1 ( Fig. 7f ). As before, addition of TAR RNA increased the effect of Tat on P-TEFb activation, but this effect was lost when the arginine-rich motif in Tat that mediates TAR binding was mutated to alanines. Mutation of cysteine residues in Tat that form two distinct zinc-fingers, one including an intermolecular zinc-finger with CycT1, diminished the stimulatory function of Tat. Likewise, an N-terminal truncation that largely omits the Tat transactivation domain almost fully abrogated Tat function. In the latter two experiments, addition of TAR even weakened the Tat effect, potentially due to the capturing of Tat from P-TEFb. Finally, we investigated the effect of human AFF4 on the activity of P-TEFb. AFF4 is a subunit of the super elongation complex that is recruited by mixed lineage leukaemia (MLL) proteins to activate the expression of MLL target genes [35] , [36] , [37] , [38] . The N-terminal 300 amino acids of AFF4 were shown to specifically interact with P-TEFb [39] , [40] . Again, the substrate specificity was tested for the consensus CTD [3] as well as serine pre-phosphorylated peptides and K7-CTD [3] . Overall, the phosphorylation profile appeared similar as for HIV-1 Tat with a considerable stimulatory effect of P-TEFb–AFF4 for the consensus CTD ( Supplementary Fig. S10 ). These results suggest similar molecular mechanisms for the stimulation of gene expression for the leukaemia-associated MLL proteins as for the viral Tat–TAR transactivation complex. Since the identification of Cdk12/Cdk13 as the human orthologues of yeast Ctk1, there has been considerable debate about the substrate specificity of RNAPII transcription regulating kinases [41] , [42] . Here we show by analytical means and western blot analysis that P-TEFb (Cdk9) specifically phosphorylates Ser5 of the hepta-repeat containing CTD. Although pre-phosphorylations of Ser7 even stimulate the catalytic activity of P-TEFb for CTD phosphorylation in the same hepta-repeat, Ser5 and Ser2 phosphorylations abrogate such double modifications. Instead, our data suggest that Ser5 and Ser2 phosphorylation of the CTD are two distinct events that are either spatially or temporally separated. Cyclin-dependent kinases Cdk1 and Cdk2 typically phosphorylate substrates of the consensus type (S/T)Px(K/R) [22] , [23] . In this motif, the amino group of the lysine residue at position +3 is involved in ionic interactions with the phospho-threonine moiety within the T-loop activation segment of the kinase [22] . Following this recognition principle, phosphorylation of Ser5 by P-TEFb assigns Tyr1 a central role in the S 5 PSY 1 sequence motif. The aromatic tyrosine is indeed the most peculiar moiety in the hepta-repeats of otherwise low sequence complexity containing another three serines, two prolines and one threonine each. The tyrosine may thus account for the kinase–substrate specificity seen here for P-TEFb that secures exactly one phosphorylation per CTD repeat. The position +2 in this connotation, which can be serine, phospho-serine or lysine, instead seems less decisive but a negative charge appears to be beneficial. The stimulatory effect of Ser7 pre-phosphorylation for priming of the CTD as P-TEFb substrate gets even more accentuated as all other phospho-modifications ascribed to the CTD (pTyr1, pSer2, pThr4 and pSer5) abrogate its subsequent phosphorylation by P-TEFb. Phosphorylation of Ser2 in the context of a pSer5 mark making an S 2 PTpS 5 recognition motif could indeed be challenging for any cyclin-dependent kinase as the presence of a double negatively charged phospho-serine at a position where typically a basic lysine or arginine resides may lead to electrostatic repulsion. In fact, it remains to be shown that such pSer2/pSer5 double phosphorylation marks exist in a single CTD hepta-repeat. The combinations of various phosphorylations in either one or two neighbouring hepta-repeats create the possibility for an additional layer of recognition specificity to mediate transcriptional regulation. Most simply, regions of Ser5 and Ser2 phosphorylation are spatially separated on the CTD, creating thus functional islands. Alternatively, stringent Ser5 dephosphorylation by phosphatases such as Rtr1 or Fcp1 in yeast [43] , [44] is required in order to render Ser2 phosphorylation possible. A recent study has indeed identified that the human RPAP2 phosphatase specifically recognizes Ser7 phosphorylation marks on the CTD to facilitate Ser5 dephosphorylation [45] . In a similar line of argument, a universal RNAPII CTD cycle along genes has been proposed, which is orchestrated by complex interplays between kinases, phosphatases and proline isomerases [46] . The determination of the minimal distances required between the two general phosphorylation marks Ser5 and Ser2 and their possible combinations with other modifications such as pSer7 might therefore be a key step in the understanding of CTD interacting proteins that recognize different phospho-isoforms during the transcription cycle [47] , [48] , [49] , [50] . Kinetic measurements with partially phosphorylated CTD substrates revealed a higher activity of P-TEFb for N-terminal progression on the periodic template compared with C-terminal progression. This might suggest a consecutive mechanistic behaviour of the enzyme with respect to pre-existing Ser5 phosphorylations. Interestingly, it was shown that an acidic motif following the last hepta-repeat of the 52 human repeats is important for its stability [51] . The ten C-terminal residues, ISPDDSDEEN, of human Rpb1 could in fact resemble an additional repeat pre-phosphorylated at positions Ser5 or Ser7 that might initiate modification of the preceding repeat. From inhibition and activation experiments performed with Hexim1 and HIV-1 Tat, respectively, we found no contributions of CycT1 to the P-TEFb-specific CTD substrate recognition. This result differs from studies of budding yeast cyclins [52] or the Cdk2/CycA complex and the substrate recognition site on CycA, which was identified to interact with the RxL motif of the substrate Cdc6 about 20 residues downstream of the phosphorylation site [22] . The corresponding surface patch on the first cyclin box repeat of CycT1 is covered both by P-TEFb-activating factors, such as Tat [33] , [53] , and by inhibitory factors, such as Hexim [30] , [31] , which do not directly contribute to substrate binding as shown here. However, co-factors of P-TEFb as shown for AFF4 of the super elongation complex could stimulate its catalytic activity or might potentially even change its substrate recognition profile. Likewise, spatial constraints in the transcription active complex could induce a processive phosphorylation mechanism, leading to continuous modification pattern on the CTD hepta-repeats. It is suggested that different combinations of Ser2, Ser5 and Ser7 phosphorylations as well as proline isomerization constitute a 'CTD code', which orchestrates transcription with pre-mRNA processing, histone modification and spliceosomal subunit arrangements [3] , [4] , [5] , [6] , [54] . The unexpected finding that P-TEFb is a Ser5 CTD kinase with a preference for Ser7 pre-phosphorylations to generate Ser5/Ser7 double-phosphorylation marks requires further structural and functional investigations on the multifaceted CTD phosphorylation patterns and their corresponding recognitions. These findings are reminiscent to observations in fission yeast where initial phosphorylation of the CTD by the kinase Mcs6 of TFIIH stimulates subsequent phosphorylation by P-TEFb, possibly to couple elongation and capping of select pre-mRNAs [55] . Likewise, the cyclin-dependent kinase Bur1/Bur2, which is the budding yeast orthologue of human Cdk9, was shown to directly stimulate Ser5 and indirectly Ser2 phosphorylation by Ctk1 during transcriptional elongation [56] . Other CTD-modifying enzymes, such as the two recently identified Cdk12 and Cdk13 kinases [41] , [42] , may additionally contribute to the variety and spatial or temporal preferences of CTD phosphorylations. The high susceptibility of Cdk9/P-TEFb for negatively charged substrates demonstrated in continuous phosphorylation imprints of every single CTD hepta-repeat, is indeed remarkable and might be a unique property of CTD-modifying kinases that are involved in the regulation of transcription. Cloning of expression plasmids and protein production The coding gene for full-length Cdk9 (1–372) was cloned into pFastBac HTb (Invitrogen) using Nco I/ Eco RI restriction sites. The bacmid for transfection of Sf 21 insect cells was obtained using the Bac-to-Bac expression system following the manufacturer's instructions (Invitrogen). His-Cdk9 was expressed in Sf 21 cells for 3 days at 27 °C by infecting cells with a third amplification Cdk9 baculovirus at 1:30 to 1:50 ratios. CycT1 (1–272) was expressed in Escherichia coli BL21(DE3) cells as described previously [57] . The heterodimeric P-TEFb complex was reconstituted by addition of purified CycT1 to the resuspended Cdk9 cells. The complex was purified using a Ni-NTA column followed by gel filtration on a Superdex 200 (16/60) column at 4 °C. Pure protein was concentrated, aliquoted and flash-frozen in liquid nitrogen. Genes encoding Hexim1 (164–359), Hexim1 (194–359), Hexim1 (207–359), Hexim1 (255–359) and Hexim1 (1–254) were cloned into pProEx-HTa containing an N-terminal hexahistidine tag. Genes for full-length Hexim1, Hexim1 (200–359) and Hexim mutants were cloned into pGEX-4T1 TEV introducing an N-terminal Glutathion-tag. Proteins were expressed in E. coli BL21(DE3) cells after addition of 0.1 mM isopropyl-β-D-thiogalactoside. Expression was carried out for 3–4 h at 30 °C or for 16 h at 20 °C. Proteins were purified using Ni-NTA or glutathione-affinity chromatography and size exclusion chromatography. The GST-tag was cut off by TEV-cleavage and removed through further purification on a gel filtration column connected to a GSH column, similarly as described [58] , [59] . HIV-1 wild-type Tat 1-86, Tat mutants C22A and C22A/C37A, mutation of the arginine-rich motif to alanine and N-terminal truncation 35–86, and HIV-1 TAR (encompassing 29 nucleotides) were prepared as recently described [31] , [57] . 7SK RNA either as full-length molecule or as 5′-end 66-mer hairpin loop was transcribed in vitro by the T7 polymerase system as described [58] . Human AFF4 1-326 was expressed as GST fusion protein from a codon-optimized expression plasmid and purified following standard procedures. Full-length Cdk9 and Cyclin T1 were purchased from ProQinase (Freiburg) at a concentration of 0.168 μg μl −1 . Similarly, Cdk7 was purchased from ProQinase as a trimeric complex containing Cdk7/CycH/MAT1 at a concentration of 0.139 μg μl −1 . RNAPII CTD proteins Plasmids containing 5, 9 or 13 CTD hepta-repeats were cloned from a synthetic oligonucleotide template as GST fusion proteins into a pGEX-4T1 TEV expression vector. A CTD sequence containing lysine at position 7 throughout was cloned following a similar strategy. GST–CTDs, designated as GST–CTD [9] or GST–CTD [13] according to the number of hepta-repeats, were expressed in BL21(DE3) or BL21 codon plus RP cells after induction with 0.1 mM isopropyl-β- D -thiogalactoside for 16 h at 20 °C. Protein purification was performed using GSH-affinity chromatography and subsequent size exclusion chromatography. In addition, a GST–CTD [8] construct was cloned with the N- and C-terminal three residues of the CTD [9] template mutated to lysines. This construct was designed for better ionization properties in the ESI-MS analyses of the otherwise fully negatively charged CTD protein. Wild-type human full-length CTD containing all 52 hepta-repeats from amino-acid sequence 1,587–1,970 including the C-terminal acidic region was cloned from genomic clone RPCIB753H14141Q (Source BioScience, UK) with Nco I and Eco RI restrictions sites at the 5′ and 3′ ends, respectively. The PCR product corresponding to cDNA sequence NM_000937 was cloned into a pGEX-6P expression vector (GE Healthcare) modified with an Nco 1 site. All expression plasmids were confirmed by DNA sequencing before expression. CTD substrate peptides For quantitative phosphorylation analyses, various CTD polypeptides were purchased from Biosyntan (Berlin) with 95% purity (HPLC grade). The peptides include a consensus CTD sequence YSPTSPSYSPTSPSYSPTSPS-[PEG] 2 -RR (cons. CTD [3] ) with a calculated mass of 2,633.8 Da; a consensus CTD continuously phosphorylated at Tyr1 PSpYSPTSPSpYSPTSPSpYSPTSPS-[PEG] 2 -RR (pY1-CTD [3] ) with a calculated mass of 3,056.0 Da; a consensus CTD continuously phosphorylated at Ser2 SYpSPTSPSYpSPTSPSYpSPTSPS-[PEG] 2 -RR (pS2-CTD [3] , calculated mass 2,960.8 Da); a consensus CTD continuously phosphorylated at Thr4 SYSPpTSPSYSPpTSPSYSPpTSPSY-[PEG] 2 -RR (pT4-CTD [3] ) with a calculated mass of 3,124.0 Da; a consensus CTD continuously phosphorylated at Ser5 YSPTpSPSYSPTpSPSYSPTpSPS-[PEG] 2 -RR (pS5-CTD [3] , calculated mass 2,873.8 Da); a consensus CTD continuously phosphorylated at Ser7 YSPTSPpSYSPTSPpSYSPTSPpSY-[PEG] 2 -RR (pS7-CTD [3] , calculated mass 3,037.0 Da); a consensus CTD phosphorylated at the N-terminal Ser5 position YSPTpSPSYSPTSPSYSPTSPS-[PEG] 2 -RR (pS5-N-CTD [3] , calculated mass 2,713.9 Da); a consensus CTD phosphorylated at the C-terminal Ser5 position SYSPTSPSYSPTSPSYSPTpSPS-[PEG] 2 -RR (pS5-C-CTD [3] , calculated mass 2,800.9 Da); and a CTD containing lysines at position 7 as found in distal CTD repeats YSPTSPKYSPTSPKYSPTSPK-[PEG] 2 -RR (K7-CTD [3] , calculated mass 2,757.1 Da). Peptides were dissolved in 50 mM HEPES, pH 7.5, to a stock concentration of 5 mM. CTD peptides were marked at the C-terminus with a double arginine motif separated by a polyethylene glycol spacer for better ionization properties in the ESI-MS experiments and for increased transfer rates in the radioactive filter-binding assay. Kinase assays using recombinant P-TEFb Radioactive kinase reactions (typically 35 μl) were carried out with recombinant highly purified proteins, using a standard protocol similarly as described [60] . P-TEFb (0.1 μM) was pre-incubated with GST–CTD (100 μM) of multiple repeats and Hexim proteins for 10 min at room temperature in kinase buffer (50 mM HEPES, pH 7.6, 34 mM KCl, 7 mM MgCl 2 , 2.5 mM dithiothreitol, 5 mM β-glycerol phosphate, 0.5 mM Na 3 VO 4 ). Cold ATP (100 μM) and 0.5 μCi [ 32 P]-γ-ATP were added and the reaction mixture incubated for 10 min at 30 °C at 300 r.p.m. For each reaction, two aliquots, 15 μl each, were spotted onto P81 Whatman paper squares and the reaction stopped by immediately immersing the paper in 0.75% (v/v) phosphoric acid. Paper squares were washed three times for 5 min with 0.75% (v/v) phosphoric acid, with at least 5 ml washing solution per paper. Radioactivity was counted in a Beckmann Scintillation Counter (Beckman Coulter) for 1 min. Typically, three experiment series were performed at different days with at least two independent measurements. Mass spectrometry analyses Peptide and protein masses were determined by liquid chromatography-electrospray ionization-mass spectrometry using an Agilent 1100 chromatography system and an LCQ Advantage MAX (Finnigan) mass spectrometer operating in positive ion mode. Proteins were applied onto an Vydac RP-C4 column (Grace) at 20% buffer B (CH 3 CN with 0.08% trifluoroacetic acid) in buffer A (H 2 O plus 0.1% TFA) and eluted with a gradient from 20–80% buffer B at a flow rate of 1 ml min −1 . Peptide samples were loaded onto the column at 5% buffer B and eluted with a gradient from 5–80% buffer B. Data evaluation was performed with the Xcalibur, MagTran and Bioworks software packages. Isothermal titration calorimetry Thermodynamic parameters of the Hexim–P-TEFb and the Hexim–CycT1 interactions were determined by ITC using either an iTC 200 or VP-ITC calorimeter (MicroCal). P-TEFb and CycT1 proteins were thermostated in the measurement cell and titrated with approximately tenfold higher concentrated Hexim proteins. Measurements with P-TEFb were carried out in two different buffers with buffer A containing 50 mM HEPES, pH 7.6, 500 mM NaCl, 10% (v/v) glycerol, 5 mM β-mercaptoethanol (high salt buffer) and buffer B containing 50 mM HEPES, pH 7.6, 250 mM NaCl, 5% (v/v) glycerol, 5 mM β-mercaptoethanol (low salt buffer). The change in heating power was observed until equilibrium was reached before the next injection was started. The data were evaluated using the manufacturer's analysis software. Western blot analysis For western blot analysis, 10 μM of human full-length GST–CTD was incubated at 30 °C with 0.04 μM P-TEFb in presence or absence of 0.4 μM Tat. Reactions were started by addition of 3 mM ATP and stopped at indicated time points by adding SDS-loading buffer to the reaction. For Coomassie staining, 1 μg of GST–CTD from the reaction mix was loaded per lane on 12% SDS–PAGE gel. For western blot analysis, 0.1 μg of GST–CTD from the reaction mix was loaded per lane on 12% SDS–PAGE gel, transferred onto nitrocellulose membrane (Whatman) and processed further by standard western-blotting protocols. For these assays, a 1:50 (α-pSer2), 1:1,000 (α-pSer5) or 1:200 (α-pSer7) dilution of primary rat IgG and 1:10,000 dilution of secondary HRP anti-rat IgG (Santa Cruz, sc-2964) antibodies were used. The anti-phospho-CTD antibodies were a kind gift from Dirk Eick, Munich. Quantitative determination of P-TEFb activity by HPLC analysis For determination of P-TEFb-mediated substrate modifications, 13-mer CTD substrate peptides were designed with either Ser2 or Ser5 residues at its centre. CTD substrate peptides were incubated at 0.25 mM concentration for 5 h at 30 °C with 0.2 μM P-TEFb in presence of 3 mM ATP. Reactions were analysed by HPLC on a Prontosil (Bischoff Chromatography) 120-5-C18 column (250×4.6 mm 2 ) using a Beckman Coulter System Gold consisting of a 126 Solvent Module and a 168 Detector set at a wavelength of 214 nm. Peptide samples were applied at a flow rate of 1 ml min −1 at 5% buffer B (CH 3 CN with 0.08% TFA) in buffer A (H 2 O plus 0.1% TFA) and eluted in a 15 min linear gradient from 5–45% buffer B. Peak fractions were collected and masses determined by liquid chromatography-electrospray ionization-mass spectrometry using an Agilent 1100 chromatography system and an LCQ Advantage MAX (Finnigan) mass spectrometer operating in positive and negative ion mode. How to cite this article: Czudnochowski, N. et al . Serine-7 but not serine-5 phosphorylation primes RNA polymerase II CTD for P-TEFb recognition. Nat. Commun. 3:842 doi: 10.1038/ncomms1846 (2012).